Enolate chemistry with anion–π interactions Anion–π interactions occur on the surface of π-acidic aromatic planes with positive quadrupole moments. Their ability to contribute to the binding and transport of anions has been demonstrated recently. However, their ability to stabilize anionic reactive intermediates and transition states remains essentially unexplored. This situation is contrary to the recognized importance of the complementary cation–π interactions to catalyse most important reactions in biology and chemistry. In this report, we provide direct experimental evidence that already single unoptimized anion–π interactions can stabilize enolates by almost two p K a units. The addition of these anion-π-stabilized reactive enolate intermediates to enones and nitroolefins occurs with transition-state stabilizations of up to 11 kJ mol −1 , and anionic cascade reactions accelerate on π-acidic surfaces. These findings are significant because enolate chemistry is central in chemistry and biology, and they will stimulate the use of anion-π interactions in catalysis in the broadest sense. The expansion of the collection of tools in hand to create molecular functional systems is of highest importance [1] . Hydrogen bonds, ion pairing and hydrophobic, π–π and cation–π interactions can be considered as the basic set of interactions between and within molecules. Recent developments with ion-pairing catalysis nicely illustrate how the clever use of already moderately innovative interactions can rapidly change a field to an entirely unpredicted extent [2] , [3] . Pertinent anion transport experiments have identified anion–π interactions [1] , [4] and halogen bonds [5] , [6] as promising candidates to contribute to the acceleration of transformations with anionic transition states. Anion–π interactions [7] , [8] , [9] , [10] , [11] , [12] , [13] , [14] , [15] , [16] , [17] , [18] , [19] , [20] , [21] , [22] , [23] , [24] are particularly intriguing because the complementary cation–π interactions are essential in biocatalysis [25] , [26] and are increasingly used in organocatalysis [25] , [27] , [28] . In sharp contrast, anion–π interactions are essentially unexplored in catalysis [23] , [24] . This is understandable because standard aromatic rings have negative quadrupole moments and are thus π-basic. Their electron-rich surfaces originate from the delocalized π-cloud of electrons below and above the plane. Naturally, they can attract cations [25] , [26] , [27] , [28] . To attract anions, the negative quadrupole moment of π-basic aromatics has to be inverted. This is possible with the introduction of strongly electron-withdrawing substituents [1] , [4] , [7] , [8] , [9] , [10] , [11] , [12] , [13] , [14] , [15] , [16] , [17] , [18] , [19] , [20] , [21] , [22] , [23] , [24] . Popular examples are hexafluorobenzene or 2,4,6-trinitrotoluene. Naphthalenediimides (NDIs) have been identified as privileged platforms to explore anion–π interactions because their intrinsic quadrupole moment is very high, and the introduction of withdrawing substituents provides access to the strongest organic π-acids known today [1] , [23] , [24] . The possibility to bind anions on the surface of π-acidic aromatics has fascinated theoreticians and crystal engineers since about a decade [7] , [8] , [9] . However, it was not easy to confirm their functional relevance in solution [4] , [10] , [14] , [16] . It has been particularly demanding to differentiate anion–π interactions, that is the interaction of anions with the electron-deficient π-orbitals on π-acidic aromatic planes with positive quadrupole moment [7] , [8] , [9] , [10] , [11] , [12] , [13] , [14] , [15] , [16] , [17] , [18] , [19] , [20] , [21] , [22] , [23] , [24] , from other phenomena. Examples include lateral contacts with π-basic aromatics by C–H … anion or dipolar interactions [29] , or even charge-transfer type interactions, which relate to anion–π interactions as conjugate acid–base pairings do to hydrogen bonds [30] . However, as soon as transmembrane transport with anion–π interactions has finally been confirmed, it was immediately clear that they should also be capable of stabilizing anionic transition states [1] . Building on an introductory study on catalysis of the Kemp elimination with anion–π interactions [23] , [24] , we here report that anion–π interactions can accelerate the reactions that are most central in chemistry [31] , [32] and biology [33] , [34] , that is, enolate chemistry. Enolate stabilization All polyketide, terpenoid and steroid natural products originate from enolate chemistry with substrates such as malonates (for example, 1 , Fig. 1 ) or acetoacetates (below) [33] , [34] . They are privileged substrates because their conjugate bases, that is, the enolates (for example, 2 ), are stabilized by resonance with two proximal carbonyl groups. To see whether these essential enolates can be stabilized by anion–π interactions, the NDI atropisomers 3 and 4 were prepared by reacting naphthalenedianhydride with the corresponding arylamines [35] , and the resulting NDI diphenols were subjected to Williamson ether synthesis with 2-bromoethanol ( Supplementary Fig. 1 ; Supplementary Methods ). The atropisomers 3 and 4 could be readily separated by thin layer chromatography. With a rotational barrier of 109.3 kJ mol −1 , these atropisomers are conformationally stable at room temperature [36] . Esterification of syn -atropisomer 4 with malonyl chloride gave the bridged NDI 5 . In the 1 H nuclear magnetic resonance (NMR) spectrum of macrocycle 5 , the resonance of the malonyl hydrogens appeared at 1.60 p.p.m. ( Fig. 1 ). Compared with the 3.38 p.p.m. for the corresponding hydrogens in diethyl malonate 1 , exposure to the ring current in NDI 5 caused an upfield shift of −1.78 p.p.m. This direct experimental evidence for the firm covalent positioning of the malonate above the π-acidic surface was of utmost importance in the context of this study, because it assured that any changes in acidity could be unambiguously attributed to the stabilization of the enolate by anion–π interactions (see below). In the dimeric macrocycle obtained with anti -atropisomer 3 , the malonyl hydrogens were not upfield shifted and thus not positioned above the π-acidic NDI surface ( Supplementary Fig. 2 ). 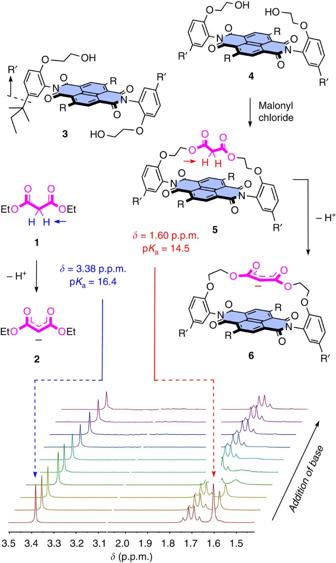Figure 1: Positioning and stabilization of enolate anions on π-acidic surfaces. 1H-NMR spectra of a 1:1 mixture of1(blue H at 3.38 p.p.m.) and5(red H at 1.60 p.p.m.) in CDCl3in the presence of increasing amounts of TMG (from bottom to top, 0.5, 1, 5, 10, 15, 20, 30, 40 and 50 equivalents) reveal that5is ΔpKa=1.9 more acidic than1, that is, a stabilization of the enolate anion on the π-acidic surface of5by ΔΔG=4.7 kJ mol−1(R=H). Figure 1: Positioning and stabilization of enolate anions on π-acidic surfaces. 1 H-NMR spectra of a 1:1 mixture of 1 (blue H at 3.38 p.p.m.) and 5 (red H at 1.60 p.p.m.) in CDCl 3 in the presence of increasing amounts of TMG (from bottom to top, 0.5, 1, 5, 10, 15, 20, 30, 40 and 50 equivalents) reveal that 5 is Δp K a =1.9 more acidic than 1 , that is, a stabilization of the enolate anion on the π-acidic surface of 5 by ΔΔ G =4.7 kJ mol −1 (R=H). Full size image In NMR titrations with 1,1,3,3-tetramethylguanidine (TMG), the resonance of the malonyl hydrogens of the bridged syn -atropisomer 5 disappeared with much less TMG than those of the diethyl malonate 1 ( Fig. 1 ). Given the known p K a =16.4 of the latter, a p K a =14.5 could be approximated for the macrocycle 5 (equation (1); Supplementary Fig. 3 ). This significantly increased acidity on a π-acidic surface, that is, Δp K a =1.9, demonstrated that the malonyl enolate anion 6 is more stable than the free enolate 2 . This increase in acidity demonstrated that the stabilization of reactive enolate intermediates 6 by anion–π interactions amounts to ΔΔ G RI =4.7 kJ mol −1 (equation (2); Fig. 2a ). With the enolate covalently positioned on the π-acidic surface in 6 and the acidity determined together with the free enolate 2 as internal control, this NMR titration provides robust experimental evidence for the stabilization of reactive enolate intermediates by anion–π interactions ( Fig. 1 ). 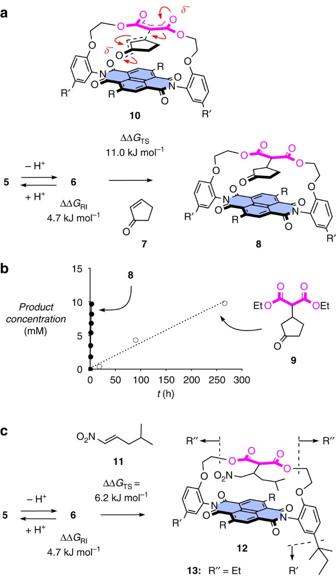Figure 2: Accelerating enolate chemistry with anion–π interactions. (a) Michael addition of macrocycle5to acceptor7. (b) Comparison of the initial velocity of the formation of Michael adduct8(filled circles) with control9(from1, empty circles) implies that anion–π interactions stabilize the anionic transition state10by ΔΔG=11.0 kJ mol−1, whereas the reactive enolate intermediate6is stabilized by ΔΔG=4.7 kJ mol−1(seeFig. 1). Conditions: 50 mM1/5, 50 mM7, 5 mM DBU, CD3CN/CDCl31:1, room temperature; linear curve fit, experiments were performed at least three times. (c) 1,4-Addition of macrocycle5to nitroolefin11with transition-state stabilization from comparison with malonate1(R=H). Figure 2: Accelerating enolate chemistry with anion–π interactions. ( a ) Michael addition of macrocycle 5 to acceptor 7 . ( b ) Comparison of the initial velocity of the formation of Michael adduct 8 (filled circles) with control 9 (from 1 , empty circles) implies that anion–π interactions stabilize the anionic transition state 10 by ΔΔ G =11.0 kJ mol −1 , whereas the reactive enolate intermediate 6 is stabilized by ΔΔ G =4.7 kJ mol −1 (see Fig. 1 ). Conditions: 50 mM 1 / 5 , 50 mM 7 , 5 mM DBU, CD 3 CN/CDCl 3 1:1, room temperature; linear curve fit, experiments were performed at least three times. ( c ) 1,4-Addition of macrocycle 5 to nitroolefin 11 with transition-state stabilization from comparison with malonate 1 (R=H). Full size image Transition-state stabilization The significance of the stabilization of enolate 6 by anion–π interactions for enolate chemistry was evaluated first with the Michael addition to enone 7 ( Fig. 2a ), a classical reaction of general interest in the community [31] , [32] , [37] . The reaction kinetics were determined by NMR spectroscopy for a 50 mM solution of 5 and 7 in CD 3 CN/CDCl 3 1:1 in the presence of 5 mM DBU (1,8-diazabicycloundec-7-ene; Supplementary Fig. 4 ). Diethyl malonate 1 was used as control without π-acidic auxiliary ( Supplementary Fig. 5 ). Linear curve fit of the formation of products 8 and 9 with time revealed that on the π-acidic surface, the Michael addition occurs 86 times faster ( Fig. 2b ; Supplementary Fig. 6 ). This significant rate enhancement demonstrated that anion–π interactions stabilize the delocalized negative charge of the transitions state 10 by ΔΔ G TS =11.0 kJ mol −1 (equations (3, 4, 5)). The general validity of this finding was evaluated with 1,4-addition of anion–π malonate 5 to nitroolefin 11 . Comparison of the velocity of the formation of product 12 with product 13 obtained with control 1 gave a transition-state stabilization of ΔΔ G TS =6.2 kJ mol −1 ( Fig. 2c ; Supplementary Figs 7–9 ). Abundant in plants, coumarins are shikimate natural products with the characteristic sweet odour of new-mown hay [34] . In chemistry, coumarins are best known as fluorescent probes and laser dyes. The synthesis of coumarin 14 from salicylaldehyde derivatives such as resorcylaldehyde 15, and esters of acetoacetate such as 16, occurs in the presence of piperidine in one step via enolate formation, Aldol condensation, elimination and transesterification ( Fig. 3a ). This reaction was selected to expand the scope of enolate chemistry with anion–π interactions towards cascade reactions. 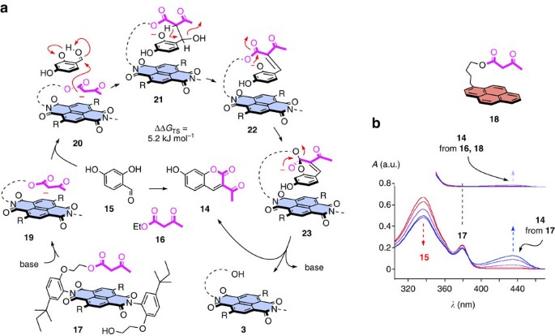Figure 3: An anionic cascade reaction on a π-acidic surface. (a) The reaction of acetoacetate17with benzaldehyde15and piperidine proceeds by enolate formation (19), aldol condensation (20), elimination (21) and transesterification (22,23) on a π-acidic surface (R=H). (b) Changes in the absorption spectra of the reaction mixture with increasing reaction time (increasing with increasing absorption of coumarin14at 435 nm). In-scale inset: same with16(or18) instead of17. Conditions: 100 mM16–18, 300 mM15, 10 mM piperidine, EtOH/CHCl31:1, room temperature. Figure 3: An anionic cascade reaction on a π-acidic surface. ( a ) The reaction of acetoacetate 17 with benzaldehyde 15 and piperidine proceeds by enolate formation ( 19 ), aldol condensation ( 20 ), elimination ( 21 ) and transesterification ( 22 , 23 ) on a π-acidic surface (R=H). ( b ) Changes in the absorption spectra of the reaction mixture with increasing reaction time (increasing with increasing absorption of coumarin 14 at 435 nm). In-scale inset: same with 16 (or 18 ) instead of 17 . Conditions: 100 mM 16 – 18 , 300 mM 15 , 10 mM piperidine, EtOH/CHCl 3 1:1, room temperature. Full size image For this purpose, the anti -atropisomer 3 was attached as π-acidic auxiliary to acetoacetate ( Fig. 1 ). A 100 mM solution of the resulting acetoacetate 17 in EtOH/CHCl 3 1:1 was reacted with 300 mM resorcylaldehyde 15 and 10 mM piperidine at room temperature. In the absorption spectra of the reaction mixture, the formation of coumarin 14 could be followed easily by the increase of the red-shifted maximum at λ max =435 nm with increasing reaction time ( Fig. 3b ). The coumarin band was fully separated from the constant absorption of π-acidic auxiliary in acetoacetate 17 at λ max =379 nm and the decreasing maximum of the benzaldehyde substrate 15 at λ max =336 nm. Linear curve fit of the increase in product concentration with time gave an apparent second-order rate constant k app =2.39±0.07 × 10 −5 M −1 s −1 ( Supplementary Fig. 10 ). Under the same conditions, the increase of the coumarin band was much slower when acetoacetate 16 without π-acidic auxiliary was used. The k app =3.00±0.16 × 10 −6 M −1 s −1 obtained for 16 demonstrated that the π-acidic surface in 17 caused a rate enhancement of k rel =8.0. This corresponded to a transition-state stabilization of ΔΔ G TS =5.2 kJ mol −1 by anion–π interactions. Acetoacetate substrates were also attached to the π-basic pyrenebutanol. For interactions on the aromatic surface, a flexible, adaptable alkyl linker as in 18 should be slightly better than the aromatic linker in 17 , although their influence should overall be negligible [24] . However, coumarin formation with cation–π control 18 was about as slow as with ethyl acetoacetate 16 ( Supplementary Fig. 10 ). The insignificant rate enhancements found with π-basic surfaces indicated that contributions from the aromatic interactions other than anion–π interactions are negligible (for example, π–π interactions with substrate 15 or cation–π interactions with iminium intermediates [27] , [38] ). In any case, the involvement of iminium intermediates is unlikely here because the aldehyde acceptors in substrate 15 are already activated by hydrogen bonding to the hydroxyl group in the ortho position. These considerations implied that the significant rate enhancement achieved on the π-acidic surface in acetoacetate 17 originates indeed from the stabilization of a series of classical anionic intermediates and transition states with anion–π interactions, beginning with an enolate 19 (compare 6 , Fig. 1). In the following aldol condensation in 20 , the negative charge moves from the enolate over to the phenolate in 21 . After completion of the Knoevenagel condensation with a dehydration, the cascade process continues with an intramolecular transesterification in 22 with the likely stabilization of the classical anionic tetrahedral intermediate of a nucleophilic substitution on a carbonyl group, and the activation of the unfavourable anionic leaving group in 23 on the π-acidic surface to ultimately afford coumarin 14 and the anti -NDI diol 3 ( Fig. 3a ). In this report, we demonstrate that anion–π interactions can stabilize the most important anionic reactive intermediates and transition states in chemistry [31] , [32] and biology [33] , [34] . Enolates, the initial reactive intermediate of all these transformations, can be stabilized by ΔΔ G RI =4.7 kJ mol −1 on isolated, unoptimized π-acidic surfaces, thus increasing the acidity of the conjugate enols by Δp K a =1.9. From enolate intermediates, unoptimized anion–π interactions can stabilize the anionic transition state of their addition to enone and nitroolefin acceptors by up to ΔΔ G TS =11.0 kJ mol −1 , or accelerate anionic cascade transformations into coumarin dyes, a process that covers Aldol condensation, elimination and transesterification. Since it is understood that catalysis in its broadest sense is defined as transition-state stabilization [39] , [40] , the use of anion–π interactions in covalent auxiliaries [41] was preferable to secure direct experimental evidence with maximal precision and minimal ambiguity based on the 1 H NMR spectra in Fig. 1 . Turnover, already demonstrated with the Kemp elimination [23] , [24] , was irrelevant for the objective of this study [39] , [40] . Previous results indicate that further π-acidification will significantly increase transition-state stabilization [1] , [4] , [23] , [24] . Core-substituted analogues (R≠H, Fig. 1 ) [1] , [23] , [24] , [42] as well as tweezers and macrocycles [1] , [4] , [21] are currently being prepared to elaborate on these expectations and initiate studies on asymmetric enolate chemistry [31] , [32] , [42] . Synthesis Malonate 5 and acetoacetates 17 and 18 were accessible in a few synthetic steps ( Supplementary Fig. 1 ; Supplementary Methods ). Spectroscopic data of analytically pure material were consistent with the proposed structures ( Supplementary Figs 11–19 ; Supplementary Methods ). 5 : TLC (CH 2 Cl 2 /acetone 40:1): R f 0.43; mp: 338–339 °C; IR (neat): 2,962 (w), 1,714 (m), 1,676 (s), 1,505 (m), 1,343 (s), 1,249 (s), 1,142 (m), 766 (m); 1 H NMR (400 MHz, CDCl 3 ): 8.79 (s, 4H), 7.38 (dd, 3 J (H,H)=8.6 Hz, 4 J (H,H)=2.3 Hz, 2H), 7.29 (d, 4 J (H,H)=2.3 Hz, 2H), 7.04 (d, 3 J (H,H)=8.6 Hz, 2H), 4.10–4.07 (m, 4H), 4.04–4.01 (m, 4H), 1.61 (q, 3 J (H,H)=7.4 Hz, 4H), 1.51 (s, 2H), 1.27 (s, 12H), 0.72 (t, 3 J (H,H)=7.4 Hz, 6H); 13 C NMR (101 MHz, CDCl 3 ): 165.3 (s), 162.9 (s), 150.7 (s), 144.7 (s), 131.4 (d), 128.2 (d), 127.8 (d), 127.2 (s), 127.0 (s), 125.4 (s), 116.2 (d), 68.0 (t), 63.9 (t), 38.1 (t), 37.7 (s), 37.1 (t), 28.4 (q), 9.2 (q); mass spectrometry (MS) (electrospray ionization (ESI), +ve): 747 (100, [M+H] + ); high-resolution MS (ESI, +ve) calculated for C 43 H 42 O 10 N 2 : 747.2912, found: 747.2908. 17 : TLC (CH 2 Cl 2 /acetone 25:1): R f 0.49; mp: 150–151 °C; IR (neat): 2,963 (w), 1,713 (s), 1,671 (s), 1,510 (m), 1,345 (s), 1,245 (s), 1,200 (m), 769 (s); 1 H NMR (400 MHz, CDCl 3 ): 8.79–8.71 (m, 4H), 7.36 (dd, 3 J (H,H)=8.7, 2.2 Hz, 2H), 7.18–7.14 (m, 2H), 7.02–6.93 (m, 2H), 4.25–4.18 (m, 2H), 4.17–4.11 (m, 4H), 3.14 (s, 2H), 2.03 (s, 3H), 1.58 (q, 3 J (H,H)=7.4 Hz, 4H), 1.24 (s, 12H), 0.72–0.67 (m, 6H); 13 C NMR (101 MHz, CDCl 3 ): 200.0 (s), 166.7 (s), 163.1 (s), 162.6 (s), 151.3 (s), 151.1 (s), 143.2 (s), 143.0 (s), 131.4 (d), 131.1 (d), 128.1 (d), 128.0 (d), 127.7 (d), 127.5 (s), 127.5 (s), 127.3 (s), 127.0 (s), 123.2 (s), 123.0 (s), 113.1 (d), 112.5 (d), 70.1 (t), 66.5 (t), 63.1 (t), 60.8 (t), 49.6 (t), 37.5 (s), 37.5 (s), 37.0 (t), 30.0 (q), 28.4 (q), 9.2 (q); MS (ESI, +ve): 763 (100, [M+H] + ); high-resolution MS (ESI, +ve) calculated for C 30 H 41 N 2 O 5 : 509.3009, found: 509.3010. Enolate stabilization To a solution of 1 (20 mM) and 5 (20 mM) in CDCl 3 were added 0.5, 1, 5, 10, 15, 20, 30, 40 and 50 equivalents of TMG as a base at room temperature (rt). 1 H NMR spectra were recorded after every addition ( Fig. 1 ). The ratio between the conjugate bases 2 and 6 and the acids 1 and 5 were determined from the integration of the indicative signals. The ratio [ 6 ]/[ 5 ] was plotted against the ratio [ 2 ]/[ 1 ], and the K a of 5 was determined from linear curve fitting to equation (1) ( Supplementary Fig. 3 ). Equation (2) gave the stabilization of the reactive enolate intermediate. Transition-state stabilization for conjugate addition Solutions of substrates S ( 5 , 1 , 50 mM), 7 (50 mM) and DBU (5 mM) were prepared in CD 3 CN/CDCl 3 1:1 at rt. 1 H NMR spectra were recorded around every 0.5 h and the concentration of the products P ( 8 , 9 ) was determined from the integration of pertinent resonances against internal standards. Concentrations of the products P were plotted against time, and the initial velocities were determined from the linear fitting ( Fig. 2b ). Apparent second-order rate constants were determined from equation (3). Rate enhancements k rel were calculated from equation (4). Transition-state stabilizations ΔΔ G TS were approximated by equation (5). The addition of malonates 5 and 1 to nitroolefin 11 (all 20 mM) was accomplished analogously in CD 3 CN/CDCl 3 1:1, at rt, in the presence of TMG (2 mM). Transition-state stabilization for coumarin synthesis Solutions of substrate S ( 16 , 17 and 18 , 100 mM), 15 (300 mM) and piperidine (10 mM) were prepared in EtOH/CHCl 3 1:1 at RT. Ultraviolet–visible spectra were recorded around every 2 h and the concentrations of the product 14 were determined from the absorption. The solvent used for ultraviolet–visible spectra was EtOH/CHCl 3 /Triethylamine 1:1:0.05. Triethylamine was used to fully deprotonate the product. Data analysis was as described above (equations (3, 4, 5)). How to cite this article: Zhao, Y. et al. Enolate chemistry with anion–π interactions. Nat. Commun. 5:3911 doi: 10.1038/ncomms4911 (2014).